Postsynaptic current bursts instruct action potential firing at a graded synapse Nematode neurons generally produce graded potentials instead of action potentials. It is unclear how the graded potentials control postsynaptic cells under physiological conditions. Here we show that postsynaptic currents frequently occur in bursts at the neuromuscular junction of Caenorhabditis elegans . Cholinergic bursts concur with facilitated action potential firing, elevated cytosolic [Ca 2+ ] and contraction of the muscle whereas GABAergic bursts suppress action potential firing. The bursts, distinct from artificially evoked responses, are characterized by a persistent current (the primary component of burst-associated charge transfer) and increased frequency and mean amplitude of postsynaptic current events. The persistent current of cholinergic postsynaptic current bursts is mostly mediated by levamisole-sensitive acetylcholine receptors, which correlates well with locomotory phenotypes of receptor mutants. Eliminating command interneurons abolishes the bursts whereas mutating SLO-1 K + channel, a potent presynaptic inhibitor of exocytosis, greatly increases the mean burst duration. These observations suggest that motoneurons control muscle by producing postsynaptic current bursts. Graded synapses transmit information encoded by presynaptic neurons or sensory receptor cells that do not fire action potentials (APs). They have been found in many species, including mammals, and contribute to diverse sensory and locomotory functions [1] , [2] , [3] , [4] , [5] , [6] , [7] . A hallmark of graded synapses is that the presynaptic cell produces graded outputs depending on the strength of stimuli received by the cell. However, properties of the postsynaptic current (PSC) underlying physiological responses are poorly characterized because the observed PSCs are usually evoked by artificial stimulation of the presynaptic cell (for example, current injection, optogenetic activation, ATP perfusion and high [K + ] o ) [1] , [2] , [3] , [5] , [6] , [7] , [8] . A description about the properties of physiological PSCs is potentially of important value to understanding how presynaptic signals control postsynaptic responses at graded synapses in vivo . C. elegans is often used as a model system for interrogating the neural circuits of sensory and motor functions. C. elegans neurons do not fire classical sodium or calcium APs. Instead, they generate graded or bistable potentials [7] , [9] , [10] , suggesting that synaptic transmission is likely graded or has other unusual properties. Recent studies show that optogenetic stimulation of presynaptic neurons causes PSCs with the peak amplitude as a function of stimulus strength [5] , [6] , [7] , which is consistent with graded synaptic transmission. However, the optogenetically evoked PSCs might be distinct from those occurring under physiological conditions because optogenetic stimuli are applied often at a saturating strength [5] , [6] , [7] , and are complicated by the fast inactivation property of channelrhodopsin-2 (ChR2) [11] , [12] . C. elegans body-wall muscle cells fire all-or-none APs [13] , [14] , whereas their innervating motoneurons likely produce graded signals [5] , which resembles the first synapse in mammalian auditory system (between hair cells and cochlear nerves) and the second synapse in mammalian visual system (between bipolar cells and ganglion cells). The present study reveals that graded transmission at the neuromuscular junction (NMJ) of worms is encoded by PSC bursts. The functional similarities between the C. elegans NMJ and some other graded synapses described above suggest that the use of PSC bursts to control postsynaptic cells likely occurs in some other graded synapses as well. PSC bursts occur concurrently in neighbouring muscle cells During our recording of endogenous PSCs at the C. elegans NMJ, the worm frequently sways its head and tail, and shows muscle contractions, suggesting that some of the endogenous PSCs might represent signals controlling muscle tension. We reasoned that any PSCs important to muscle activity should occur concurrently in neighbouring muscle cells because these cells contract and relax concertedly to produce the sinusoidal locomotion. To identify such PSC events, we recorded endogenous PSCs from a pair of neighbouring muscle cells, and scrutinized the recording traces for concurrent events that are potentially important to muscle activity. The L2R2 pair of ventral muscle cells at the same position along the longitudinal body axis ( Fig. 1a ) was chosen for the analysis because they are controlled by the same motoneurons [15] , [16] but have little electrical coupling [17] , [18] . We noticed that PSCs occurred both sporadically and in bursts. Interestingly, PSC bursts of relatively long duration (>3 s) always concurred in both cells ( Fig. 1b ), which raised the possibility that they represent physiological signals controlling muscle tension. 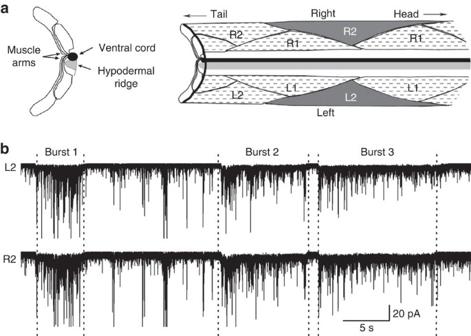Figure 1: PSC bursts occur concurrently in a pair of neighbouring body-wall muscle cells. (a) Diagrams showing the anatomy of ventral body-wall muscles. The left panel is a cross section of the muscles shown on the right. Two muscle strips known as quadrants run beside the ventral nerve cord. Muscle cells in the right quadrant are designated as R1 and R2 whereas those in the left quadrant as L1 and L2. One L2R2 cell pair was highlighted. (b) Voltage-clamp recording showing that PSC bursts happened concurrently in the L2R2 cell pair. The holding potential was −60 mV. Extracellular solution I and pipette solution I were used. Only those PSC bursts meeting our criterion (an apparent increase in PSC frequency with a baseline shift lasting>3 s) are labelled as bursts. Figure 1: PSC bursts occur concurrently in a pair of neighbouring body-wall muscle cells. ( a ) Diagrams showing the anatomy of ventral body-wall muscles. The left panel is a cross section of the muscles shown on the right. Two muscle strips known as quadrants run beside the ventral nerve cord. Muscle cells in the right quadrant are designated as R1 and R2 whereas those in the left quadrant as L1 and L2. One L2R2 cell pair was highlighted. ( b ) Voltage-clamp recording showing that PSC bursts happened concurrently in the L2R2 cell pair. The holding potential was −60 mV. Extracellular solution I and pipette solution I were used. Only those PSC bursts meeting our criterion (an apparent increase in PSC frequency with a baseline shift lasting>3 s) are labelled as bursts. Full size image Cholinergic and GABAergic PSC bursts have opposite effects If PSC bursts were indeed physiologically important, they should be associated with changes in muscle activity. The PSCs shown in Fig. 1b were recorded at −60 mV holding potential in the presence of high [Cl − ] in the pipette solution. As a result, all PSCs appeared as inward current events although they were mediated by two different types of receptors: acetylcholine (ACh) receptor and γ-aminobutyric acid (GABA) receptor. To assess the potential physiological roles of cholinergic and GABAergic motoneurons, we used experimental conditions to isolate cholinergic and GABAergic PSCs and analysed temporal relationships between PSC bursts and muscle APs or Ca 2+ transients. ACh receptor-mediated PSCs were recorded using pipette and extracellular solutions with the chloride equilibrium potential equal to the holding potential (−60 mV). GABA receptor-mediated PSCs were recorded by holding the membrane potential at −10 mV and using different pipette and extracellular solutions [14] , [19] , which allowed muscle to fire APs at a much higher rate, making it easier to detect an inhibitory effect of GABAergic bursts. Temporal relationships between PSC bursts and muscle APs were assessed through analysing simultaneously recorded PSCs from one cell (voltage-clamped) and APs from the other cell (current-clamped) of the L2R2 pair, where AP firing in one cell was not affected by the holding potential of the other cells ( Supplementary Fig. S1 ). The effect of PSC bursts on muscle Ca 2+ transients was assessed by recording PSCs from one cell and Ca 2+ transients from a neighbouring cell in a strain expressing GCaMP2 in body-wall muscle [13] . This approach was appropriate because Ca 2+ transients are synchronous in neighbouring muscle cells [18] . Spontaneous PSC bursts mediated by ACh receptors were frequently observed and generally concurred with facilitated muscle AP firing, Ca 2+ transients and cell shortening ( Fig. 2a and Supplementary Movie 1 ). The total charge transfer of PSC bursts correlated positively with [Ca 2+ ] i ( r =0.86), which correlated negatively with muscle cell length ( r =0.87) ( Fig. 2b ). These observations suggest that cholinergic motoneurons cause muscle contractions by producing excitatory PSC (EPSC) bursts. It appeared that the duration of a PSC burst had to be longer than ~3 s to observe a concurrent muscle Ca 2+ transient. Interestingly, PSC bursts showing temporal correlations with Ca 2+ transients were invariably associated with a persistent current ( Fig. 2 and Supplementary Fig. S2 ). To objectively analyse physiologically important PSC bursts without relying on Ca 2+ imaging, we defined a PSC burst as an apparent increase in PSC frequency with a persistent current lasting >3 s. The duration of the persistent current was used as the duration of a PSC burst throughout this study. 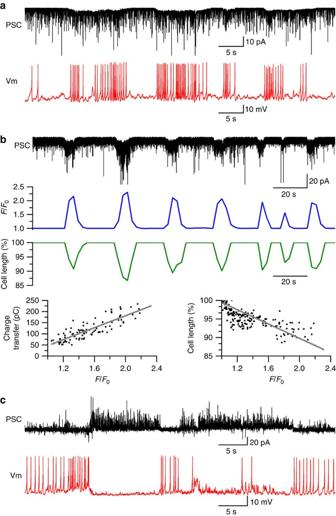Figure 2: PSC bursts instruct muscle activities. (a,b). Spontaneous cholinergic PSC bursts were associated with facilitated muscle AP firing (a), increased cytosolic [Ca2+] and shortening of muscle cells (b). Cytosolic [Ca2+] was positively correlated with the total charge transfer of endogenous PSC bursts but negatively correlated with muscle cell length. A movie of this representative experiment is shown in the supplement (Supplementary Movie 1). (c) Spontaneous GABAergic PSC bursts suppressed muscle AP firing. Cholinergic PSCs appeared as inward currents (downward deflections) whereas GABAergic PSCs appeared as outward currents (upward deflections). The traces were from a light-off period in a transgenic worm expressing ChR2 in GABAergic neurons. The holding potential was −60 mV inaandbbut −10 mV inc. The experiments ina,bwere performed with extracellular solution I and either pipette solution I (for APs) or pipette solution III (for PSCs). The experiment incwas performed with extracellular solution II and pipette solution II. Figure 2: PSC bursts instruct muscle activities. ( a , b ). Spontaneous cholinergic PSC bursts were associated with facilitated muscle AP firing ( a ), increased cytosolic [Ca 2+ ] and shortening of muscle cells ( b ). Cytosolic [Ca 2+ ] was positively correlated with the total charge transfer of endogenous PSC bursts but negatively correlated with muscle cell length. A movie of this representative experiment is shown in the supplement ( Supplementary Movie 1 ). ( c ) Spontaneous GABAergic PSC bursts suppressed muscle AP firing. Cholinergic PSCs appeared as inward currents (downward deflections) whereas GABAergic PSCs appeared as outward currents (upward deflections). The traces were from a light-off period in a transgenic worm expressing ChR2 in GABAergic neurons. The holding potential was −60 mV in a and b but −10 mV in c . The experiments in a , b were performed with extracellular solution I and either pipette solution I (for APs) or pipette solution III (for PSCs). The experiment in c was performed with extracellular solution II and pipette solution II. Full size image Spontaneous PSC bursts mediated by GABA receptors, however, were not readily observed in wild-type worms. Intriguingly, in a transgenic strain used to examine the effect of photostimulation on GABAergic PSC bursts (described later), spontaneous GABAergic PSC bursts were frequently observed during blue light-off periods (frequency: 1.17±0.13 min −1 ; duration: 8.72±0.66 s, n =9), and always associated with a suppression of AP firing ( Fig. 2c ). There was also no other microscope illumination during the recording. While the mechanism for the spontaneous occurrence of GABAergic bursts in the transgenic strain is unclear, these observations suggest that GABAergic bursts could potentially occur in intact worms. C. elegans locomotion may be modulated by the activation of stretch-sensitive channels in motoneurons or some other neurons [20] , [21] , [22] , [23] . In the present study, the head and tail of the worm were allowed to sway during the experiment, which could potentially affect PSC bursts. To determine whether this was the case, we compared the frequency and duration of cholinergic PSC bursts between wild-type worms with head and tail freely moving (Control) and those with the head and tail immobilized by gluing. We found that both the frequency and duration of PSC bursts were similar between these two groups (Control 3.05±0.40 min −1 , 7.40±0.58 s, n =8; Head and tail immobilized 3.12±0.41 min −1 , 7.73±0.53 s, n =7). PSC bursts greatly increase postsynaptic charge transfer To understand why PSC bursts were sufficient to control muscle activity, we compared properties of PSCs between intra-burst and extra-burst periods. PSCs frequently appeared as multiphasic events (two or more PSCs clustering together without returning to the baseline, Fig. 3a , middle panels), especially during PSC bursts. Multiphasic events were included for quantifying PSC frequency but excluded for quantifying PSC amplitude, charge transfer, half width, 10–90% rise time and decay time. 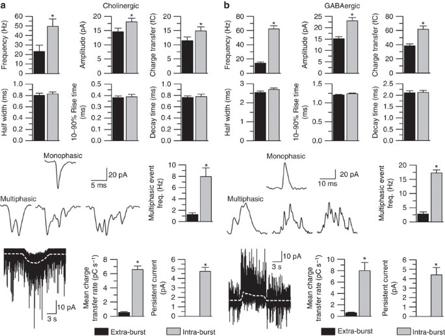Figure 3: PSC bursts are characterized by increased PSC activity and the appearance of a persistent current. Properties of cholinergic (a) and GABAergic (b) PSC bursts. Top: Comparisons of PSC frequency, mean amplitude, mean charge transfer, half-width, 10–90% rise time and decay time between intra- and extra-burst periods. The frequency was quantified from all PSCs whereas the other parameters were quantified from only monophasic PSCs. Middle: Sample monophasic and multiphasic PSCs and comparison of their frequencies between intra- and extra-burst periods. Bottom: Sample PSC bursts, and comparisons of the mean charge transfer rate and persistent current amplitude between intra- and extra-burst periods. The quantification was performed with the same data represented inFig. 2. The asterisk indicates a significant difference compared with the extra-burst period (P<0.05, pairedt-test).n=9 in bothaandb. Data are shown as mean±s.e. Figure 3: PSC bursts are characterized by increased PSC activity and the appearance of a persistent current. Properties of cholinergic ( a ) and GABAergic ( b ) PSC bursts. Top: Comparisons of PSC frequency, mean amplitude, mean charge transfer, half-width, 10–90% rise time and decay time between intra- and extra-burst periods. The frequency was quantified from all PSCs whereas the other parameters were quantified from only monophasic PSCs. Middle: Sample monophasic and multiphasic PSCs and comparison of their frequencies between intra- and extra-burst periods. Bottom: Sample PSC bursts, and comparisons of the mean charge transfer rate and persistent current amplitude between intra- and extra-burst periods. The quantification was performed with the same data represented in Fig. 2 . The asterisk indicates a significant difference compared with the extra-burst period ( P <0.05, paired t -test). n =9 in both a and b . Data are shown as mean±s.e. Full size image Statistical analyses were first performed with data of the same experimental groups as represented in Fig. 2 . Compared with extra-burst events, intra-burst PSCs showed significant increases in the mean frequency, amplitude and charge transfer but no change in the half width, 10–90% rise time and decay time ( Fig. 3a , top). There was no obvious causal relationship between the larger mean amplitude of intra-burst PSCs and the persistent current because the amplitude of intra-burst PSCs was determined from the shifted baseline ( Supplementary Fig. S2 ). The PSC burst was accompanied by a more than fivefold increase in multiphasic events ( Fig. 3a , middle). The mean charge transfer rate of PSCs (pC s −1 ) during the intra-burst period was much higher than that during the extra-burst period ( Fig. 3a , bottom). The primary contributor to the increased charge transfer rate during PSC bursts was the persistent current, which accounted for 76.5 and 53.7% of the cholinergic and GABAergic intra-burst charge transfers, respectively. The expression of GCaMP2 in muscle had no effect on extra- and intra-burst PSCs ( Supplementary Fig. S3 ). Optogenetically evoked PSCs differ from endogenous bursts Previous studies of graded synaptic transmission in C. elegans relied on optogenetic stimulation of presynaptic neurons [5] , [6] , [7] . To evaluate to what degree optogenetically evoked postsynaptic responses mimic endogenous PSC bursts, we recorded photo-evoked PSCs and APs simultaneously in the L2R2 cell pair of two strains expressing mCherry-tagged ChR2 in cholinergic and GABAergic neurons, respectively [5] . The worms were raised in either the presence or the absence of the light-sensing cofactor all- trans retinal [11] and subjected to 2-s light pulses at 30 s intervals. In worms that had been raised in retinal, photostimulation of cholinergic motoneurons evoked inward PSCs and facilitated AP firing ( Fig. 4a ) but that of GABAergic motoneurons evoked outward PSCs and inhibited AP firing ( Fig. 4b ). The rate of AP firing during the light-off period was much higher in Fig. 4b than in Fig. 4a because of the use of different pipette and extracellular solutions rather than the different holding potentials of the voltage-clamped cells ( Supplementary Fig. S1 ). In contrast, worms that had not been raised in retinal did not show any photo-evoked response ( Fig. 4a ). Similar to photo-evoked responses at a C. elegans nociceptive sensory synapse [6] , the evoked PSC at the NMJ had three prominent components, including a huge initial transient, a persistent current and an increased frequency of unitary PSC events ( Fig. 4a ). The optogenetically evoked responses differed from endogenous PSC bursts in having the additional huge initial transient, a larger persistent current and a higher PSC frequency. 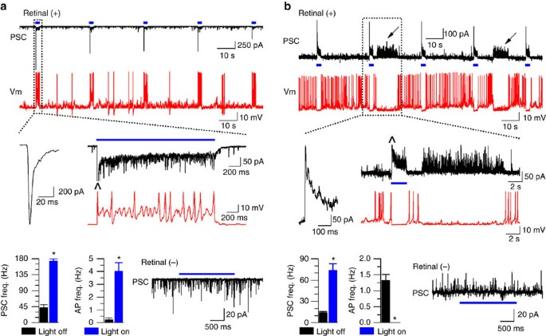Figure 4: Optogenetically evoked cholinergic and GABAergic PSCs modulate AP firing. Experiments were performed with transgenic worms expressing ChR2 in either cholinergic (a) or GABAergic (b) neurons. The worms were raised either in the presence or absence of all-transretinal as indicated. PSCs and APs were recorded simultaneously from the L2R2 cell pair. Top: Temporal relationships between evoked PSCs and muscle APs. The horizontal blue lines represent blue light pulses. The arrows mark spontaneous GABAergic PSC bursts during light-off periods. The ‘^’ sign indicates that the peak was cut off. Middle: a segment of the recording traces in the top panels (indicated by the dotted rectangle) shown at expanded scales. The initial transient current is displayed separately on the left. Bottom: comparisons of PSC and AP frequencies between light-on and light-off periods (n=8 ina;n=9 inb) and representative traces from worms that had not been raised in the presence of retinal (representative of three experiments in bothaandb). The asterisk indicates a significant difference compared with the light-off period (P<0.01, pairedt-test). The data shown inawere performed with extracellular solution I and pipette solution I whereas those shown inbwere performed with extracellular solution II and pipette solution II. Data are shown as mean±s.e. Figure 4: Optogenetically evoked cholinergic and GABAergic PSCs modulate AP firing. Experiments were performed with transgenic worms expressing ChR2 in either cholinergic ( a ) or GABAergic ( b ) neurons. The worms were raised either in the presence or absence of all- trans retinal as indicated. PSCs and APs were recorded simultaneously from the L2R2 cell pair. Top: Temporal relationships between evoked PSCs and muscle APs. The horizontal blue lines represent blue light pulses. The arrows mark spontaneous GABAergic PSC bursts during light-off periods. The ‘ ^ ’ sign indicates that the peak was cut off. Middle: a segment of the recording traces in the top panels (indicated by the dotted rectangle) shown at expanded scales. The initial transient current is displayed separately on the left. Bottom: comparisons of PSC and AP frequencies between light-on and light-off periods ( n =8 in a ; n =9 in b ) and representative traces from worms that had not been raised in the presence of retinal (representative of three experiments in both a and b ). The asterisk indicates a significant difference compared with the light-off period ( P <0.01, paired t -test). The data shown in a were performed with extracellular solution I and pipette solution I whereas those shown in b were performed with extracellular solution II and pipette solution II. Data are shown as mean±s.e. Full size image ChR2 inactivates to almost 80% within the first 100 ms of photostimulation [12] , which raised the question whether the persistent current and higher PSC frequency following the huge initial peak response were simply residual effects of the peak response. To examine this possibility, we stimulated worms with a 50-ms light pulse and compared PSC frequency at three different intervals from the beginning of the photostimulus: 500–1,000, 1,000–1,500 and 1,500–2,000 ms. The PSC frequency was similar during the three different intervals, and indistinguishable from that of the prestimulation period. Furthermore, we did not detect any persistent current ( Supplementary Fig. S4 ). These observations suggest that the initial transient did not have a long-lasting effect. Persistent currents rely on specific postsynaptic receptors As the persistent current of PSC bursts was the primary contributor to burst-associated charge transfer, it is important to identify the membrane channels carrying it. We first tested the effects of (+)-tubocurarine (TBC) and gabazine (SR-95531), which block ACh receptors and GABA receptors, respectively, in C. elegans body-wall muscle [18] , [24] . The experiments were performed with the two worm strains expressing ChR2 in cholinergic neurons and GABAergic neurons because the larger persistent current of optogenetically evoked responses made the assay more sensitive. We found that the persistent currents of cholinergic and GABAergic PSC bursts were abolished by TBC (0.5 mM) and gabazine (0.5 mM), respectively ( Fig. 5a ), suggesting that they were mediated by muscle ACh receptors and GABA A receptors. 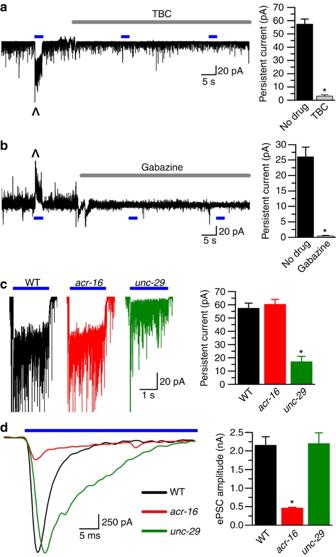Figure 5: Optogenetically evoked cholinergic and GABAergic PSC bursts depended on specific postsynaptic receptors. (a,b) Left: sample traces from worms raised in the presence of all-transretinal showing the effects of (+)-TBC (0.5 mM) and gabazine (0.5 mM) on optogenetically evoked cholinergic and GABAergic PSC bursts, respectively. The horizontal blue lines represent blue light pulses while the ‘^’ sign indicates that the peak was cut off. Right: the persistent current of evoked cholinergic (n=15) and GABAergic (n=12) bursts were abolished by TBC and gabazine, respectively. (c) The persistent current of evoked cholinergic PSC bursts was greatly decreased inunc-29(e1072)but unchanged inacr-16(ok789)compared with wild type (WT). (d) The large initial transient of evoked cholinergic PSC bursts was greatly decreased inacr-16(ok789)but unchanged inunc-29(e1072)compared with WT. Inc,d, the sample size (n) was eight for every group. The WT group is the same as that shown inFig. 4. The asterisk (*) indicates a statistically significant difference (P<0.01) compared with either the control period inaorb(pairedt-test) or the WT group incandd(one-way analysis of variance followed by Bonferronipost hoctest). Inaandb, extracellular solution I and pipette solution III were used to record cholinergic PSCs whereas extracellular solution II and pipette solution II were used to record GABAergic PSCs. Incandd, extracellular solution I and pipette solution I were used. Figure 5: Optogenetically evoked cholinergic and GABAergic PSC bursts depended on specific postsynaptic receptors. ( a , b ) Left: sample traces from worms raised in the presence of all- trans retinal showing the effects of (+)-TBC (0.5 mM) and gabazine (0.5 mM) on optogenetically evoked cholinergic and GABAergic PSC bursts, respectively. The horizontal blue lines represent blue light pulses while the ‘ ^ ’ sign indicates that the peak was cut off. Right: the persistent current of evoked cholinergic ( n =15) and GABAergic ( n =12) bursts were abolished by TBC and gabazine, respectively. ( c ) The persistent current of evoked cholinergic PSC bursts was greatly decreased in unc-29(e1072) but unchanged in acr-16(ok789) compared with wild type (WT). ( d ) The large initial transient of evoked cholinergic PSC bursts was greatly decreased in acr-16(ok789) but unchanged in unc-29(e1072) compared with WT. In c , d , the sample size ( n ) was eight for every group. The WT group is the same as that shown in Fig. 4 . The asterisk (*) indicates a statistically significant difference ( P <0.01) compared with either the control period in a or b (paired t -test) or the WT group in c and d (one-way analysis of variance followed by Bonferroni post hoc test). In a and b , extracellular solution I and pipette solution III were used to record cholinergic PSCs whereas extracellular solution II and pipette solution II were used to record GABAergic PSCs. In c and d , extracellular solution I and pipette solution I were used. Full size image ACh receptors in C. elegans body-wall muscle include a nicotine-sensitive receptor (N-AChR) and a levamisole-sensitive receptor (L-AChR). The former appears to be a homomeric complex of the ACR-16 subunit [25] , [26] whereas the latter consists of several different subunits, including UNC-29 ( [27] ). To determine which ACh receptor(s) is important, we compared amplitudes of the persistent current and the large initial transient between wild type and mutants of acr-16(ok789) and unc-29(e1072) [24] , [25] , [26] . The persistent current was decreased by ~70% in the unc-29 mutant but unchanged in the acr-16 mutant ( Fig. 5c ) whereas the initial transient was decreased by ~80% in the acr-16 mutant but unchanged in the unc-29 mutant ( Fig. 5d ). These observations, similar to those of a previous study [28] , suggest that the initial transient was mediated mainly by the N-AChR whereas the persistent current mainly by the L-AChR. Surprisingly, the PSC peak current decayed more slowly in the unc-29 mutant ( τ =12.38±1.25 ms, n =8) than wild type ( τ =4.71±0.37 ms, n =7) ( Fig. 5d ), which could have resulted from developmental changes affecting either ACh release or postsynaptic AChRs. Stimulation of command interneurons evokes bursts in muscle The large initial transient caused by optogenetic stimulation of motoneurons resembles the evoked responses caused by either optogenetic or electric stimulation of C. elegans motoneurons [5] , [29] , [30] . Its absence in endogenous PSC bursts suggested that the membrane voltage changes caused by optogenetic stimulation of motoneurons probably do not mirror endogenous voltage changes. To confirm this, we expressed ChR2 in command interneurons under the control of glr-1 (glutamate receptor subunit) promoter [31] , and recorded optogenetically evoked PSCs and APs from body-wall muscle cells. It is known that cholinergic motor neurons are controlled by command interneurons through gap junctions and chemical synapses [32] , [33] , [34] , [35] . We reasoned that the gap junctions and chemical synapses might serve as a low-pass filter to allow the occurrence of PSC bursts but not of the large initial transient upon photostimulation of command interneurons. Indeed, in worms that had been raised in retinal, photostimulation evoked PSC bursts that were qualitatively similar to endogenous PSC bursts, and sufficient for facilitating muscle AP firing ( Fig. 6a ). Control worms that had been raised in the absence of retinal showed no evoked PSC bursts ( Fig. 6c ). These observations reinforce the notion that motoneurons control body-wall muscle cells by producing PSC bursts. 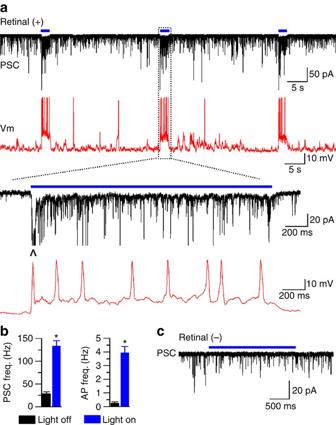Figure 6: Optogenetic stimulation of command interneurons caused postsynaptic responses resembling spontaneous PSC bursts. The experiments were performed with worms expressing ChR2 in command interneurons. The worms had been raised in either the presence or the absence of all-transretinal as indicated. (a) Sample traces showing PSCs and membrane potentials recorded simultaneously from a L2R2 cell pair of a worm raised in all-transretinal. Photo-stimuli (marked by the blue horizontal line) evoked PSC bursts, which facilitated AP firing. The ‘^’ sign indicates that the peak was cut off. (b) Comparisons of PSC and AP frequencies between light-on and light-off periods (n=7). The asterisk indicates a significant difference (P<0.01, pairedt-test). Data are shown as mean±s.e. (c) A sample trace from a worm raised in the absence of retinal showing that a photostimulus (marked by the blue horizontal line) had no effect on PSCs (representative of three experiments). The experiments were performed with extracellular solution I and either pipette solution I (for APs) or pipette solution III (for PSCs). Figure 6: Optogenetic stimulation of command interneurons caused postsynaptic responses resembling spontaneous PSC bursts. The experiments were performed with worms expressing ChR2 in command interneurons. The worms had been raised in either the presence or the absence of all- trans retinal as indicated. ( a ) Sample traces showing PSCs and membrane potentials recorded simultaneously from a L2R2 cell pair of a worm raised in all- trans retinal. Photo-stimuli (marked by the blue horizontal line) evoked PSC bursts, which facilitated AP firing. The ‘ ^ ’ sign indicates that the peak was cut off. ( b ) Comparisons of PSC and AP frequencies between light-on and light-off periods ( n =7). The asterisk indicates a significant difference ( P <0.01, paired t -test). Data are shown as mean±s.e. ( c ) A sample trace from a worm raised in the absence of retinal showing that a photostimulus (marked by the blue horizontal line) had no effect on PSCs (representative of three experiments). The experiments were performed with extracellular solution I and either pipette solution I (for APs) or pipette solution III (for PSCs). Full size image Cholinergic PSC bursts depend on command interneurons The PSC bursts could either originate in motoneurons or be triggered by higher-order neurons. To distinguish between these two possibilities, we investigated the role of command interneurons in the generation of cholinergic PSC bursts. Five pairs of command interneurons control cholinergic motoneurons through chemical synapses and gap junctions [33] . Two specific innexins, UNC-7 and UNC-9, appear to be important components of the gap junctions with mutations of either innexin causing severe locomotion defects [34] , [35] . We analysed cholinergic PSC bursts in unc-7(e5) and unc-9(fc16) mutants, which are putative nulls [36] , [37] . We found that PSC burst frequency was reduced by more than 50% in either the unc-7 or the unc-9 mutant compared with wild-type worms ( Fig. 7 ), suggesting that electrical coupling between command interneurons and motoneurons has an important role in PSC bursts. Intriguingly, the remaining PSC bursts in either mutant were longer in duration and larger in mean charge transfer rate and persistent current amplitude ( Fig. 7 ). To further assess the role of command interneurons, we recorded cholinergic PSCs in worms with the head and tail cut off by a diamond dissecting knife to eliminate all command interneurons. We did not detect any cholinergic PSC bursts in these worms ( Fig. 7 ). The absence of PSC bursts in these worms did not result from damaged motoneurons because PSCs evoked by photostimulation of motoneurons expressing ChR2 were indistinguishable between control worms (2.15±0.23 nA, n =8) and worms with head and tail cut off (2.03±0.20 nA, n =5). These observations suggest that cholinergic PSC bursts were initiated by command interneurons and/or other higher-order neurons. 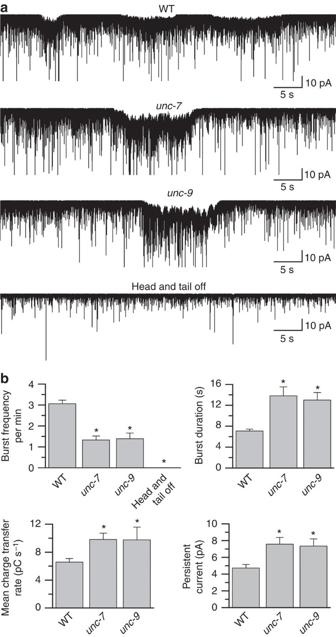Figure 7: Cholinergic PSC bursts appear to be dependent on inputs from command interneurons. (a) Sample PSC traces representing wild type (WT) (n=9),unc-7(e5)(n=7),unc-9(fc16)(n=9) and a worm with all command interneurons removed (head and tail off) (n=6). (b) Comparisons of PSC burst frequency, duration, charge transfer rate and persistent current amplitude. PSC bursts were completely absent in the head and tail off group. The asterisk (*) indicates a statistically significant difference compared with WT (P<0.05, one-way analysis of variance). Extracellular solution I and pipette solution III were used in these experiments. Data are shown as mean±s.e. Figure 7: Cholinergic PSC bursts appear to be dependent on inputs from command interneurons. ( a ) Sample PSC traces representing wild type (WT) ( n =9), unc-7(e5) ( n =7), unc-9(fc16) ( n =9) and a worm with all command interneurons removed (head and tail off) ( n =6). ( b ) Comparisons of PSC burst frequency, duration, charge transfer rate and persistent current amplitude. PSC bursts were completely absent in the head and tail off group. The asterisk (*) indicates a statistically significant difference compared with WT ( P <0.05, one-way analysis of variance). Extracellular solution I and pipette solution III were used in these experiments. Data are shown as mean±s.e. Full size image Mutation of SLO-1 K + channel increases PSC burst duration The Ca 2+ - and voltage-gated K + channel SLO-1 is a potent negative regulator of neurotransmitter release at the C. elegans NMJ [38] , [39] . To determine whether the regulatory role of SLO-1 in neurotransmitter release is reflected in PSC bursts, we compared the frequency and duration of cholinergic PSC bursts between wild type and slo-1(md1745) , a putative null mutant [38] . The worms expressing GCaMP2 in body-wall muscle cells [13] were used for these experiments so that Ca 2+ transients and PSCs could be recorded at the same time. The mean duration of PSC bursts was greatly prolonged in the slo-1 mutant compared with wild type ( Fig. 8 ), which is consistent with the inhibitory role of SLO-1 in neurotransmitter release. While the frequency of PSC bursts had no change, that of muscle Ca 2+ transients increased by >2-fold in the slo-1 mutant compared with wild type ( Fig. 8 , Supplementary Movies 2,3 ). Thus, unlike an essentially 1 to 1 ratio between cholinergic PSC bursts and muscle Ca 2+ transients in wild-type worms, the frequency of Ca 2+ transients was significantly higher than that of PSC bursts in the slo-1 mutant. slo-1 deficiency in muscle was at least partially responsible for the higher frequency of muscle Ca 2+ transients [40] . These observations suggest that SLO-1 may control synaptic strength and muscle activity through modulating PSC bursts. 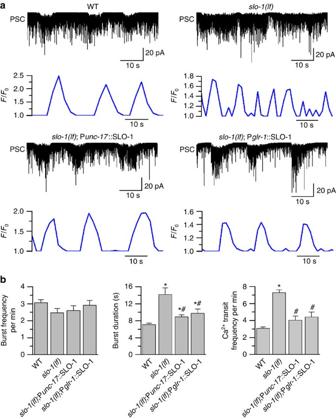Figure 8: Loss-of-function mutation of SLO-1 K+channels increases cholinergic PSC burst duration and muscle Ca2+transient frequency. (a) Sample traces of PSCs and muscle Ca2+transients representing wild type (WT) (n=9),slo-1(md1745)(n=9),slo-1(md1745)rescued in cholinergic neurons usingunc-17promoter (Punc-17) (n=7), andslo-1(md1745)rescued in command interneurons usingglr-1promoter (Pglr-1) (n=7). Ca2+transients of these representative experiments are shown inSupplementary Movies 2–5. (b) Comparisons of the frequency and duration of PSC bursts, and the frequency of Ca2+transients among the different groups. The asterisk (*) indicate a significant difference compared with WT whereas the pound sign (#) indicates a significant difference compared withslo-1(P<0.05, one-way analysis of variance with Bonferronipost hoctests). Quantitative comparisons for other parameters of intra- and extra-burst PSCs are shown inSupplementary Fig. S5. Extracellular solution I and pipette solution III were used in these experiments. Data are shown as mean±s.e. Figure 8: Loss-of-function mutation of SLO-1 K + channels increases cholinergic PSC burst duration and muscle Ca 2+ transient frequency. ( a ) Sample traces of PSCs and muscle Ca 2+ transients representing wild type (WT) ( n =9), slo-1(md1745) ( n =9), slo-1(md1745) rescued in cholinergic neurons using unc-17 promoter ( Punc-17 ) ( n =7), and slo-1(md1745) rescued in command interneurons using glr-1 promoter ( Pglr-1 ) ( n =7). Ca 2+ transients of these representative experiments are shown in Supplementary Movies 2–5 . ( b ) Comparisons of the frequency and duration of PSC bursts, and the frequency of Ca 2+ transients among the different groups. The asterisk (*) indicate a significant difference compared with WT whereas the pound sign (#) indicates a significant difference compared with slo-1 ( P <0.05, one-way analysis of variance with Bonferroni post hoc tests). Quantitative comparisons for other parameters of intra- and extra-burst PSCs are shown in Supplementary Fig. S5 . Extracellular solution I and pipette solution III were used in these experiments. Data are shown as mean±s.e. Full size image To determine whether SLO-1 functions in command interneurons or cholinergic motoneurons to regulate PSC bursts, we analysed the effects of targeted slo-1 rescue in command interneurons and cholinergic neurons by expressing wild-type SLO-1 under the control of glr-1 promoter and unc-17 promoter, respectively. We found that expression of wild-type SLO-1 in either cholinergic neurons or command interneurons largely rescued the effect of slo-1 mutation on PSC burst duration and completely rescued the effect of slo-1 mutation on muscle Ca 2+ transients ( Fig. 8 , Supplementary Movies 4,5 ). These observations suggest that SLO-1 may function in both command interneurons and motoneurons to regulate the duration of PSC bursts. We also analysed other properties of extra- and intra-burst cholinergic PSCs for the slo-1 mutant and the two targeted rescue strains as we did for wild-type worms. These analyses did not reveal any significant difference compared with wild type ( Supplementary Fig. S5 ). Therefore, the function of SLO-1 appears to be limited to regulating the duration of PSC bursts. One intriguing feature of the C. elegans NMJ is that spontaneous PSCs are observed at a very high frequency [41] . Physiological significance of the spontaneous PSCs has been unclear. The results of the present study provide compelling evidence that motoneurons control the muscle by producing PSC bursts. PSC bursts distinguish themselves from the extra-burst period by three characteristic properties: a higher PSC frequency, a larger mean PSC amplitude and a persistent current. The increased PSC frequency reflects increased presynaptic release probability. The larger PSC amplitude could be caused by a variety of factors, such as the activation of presynaptic ryanodine receptors [42] . The persistent current results from the activation of muscle ACh or GABA receptor. Previous analyses of ACh receptor mutants have shown that mutants of N-AChR show greatly decreased amplitude of evoked PSCs but are apparently normal in locomotion whereas mutants of L-AChR have essentially normal evoked PSCs but are severely sluggish [26] . The larger effect of L-AChR mutation on locomotion could be due to a much smaller persistent current resulting from the absence of the slow desensitizing L-AChR [24] , [25] , [26] . PSC bursts were associated with a more than tenfold increase in the mean charge transfer rate compared with extra-burst period. Nevertheless, the mean current flow rate during burst was still small. How could such a small current be sufficient to facilitate or inhibit muscle AP firing? Three properties of C. elegans body-wall muscle cells likely contributed to this high sensitivity, including a high membrane input resistance (~1.5 GΩ) [17] , a resting membrane potential that is close to the threshold of AP firing [13] , [14] and an intrinsic ability of firing APs [13] , [43] . Spontaneous GABAergic PSC bursts were not observed in wild-type preparations in the present study, which could be owing to the lack of presynaptic inputs to GABAergic motoneurons. GABAergic motoneurons innervating the ventral muscle are controlled by cholinergic motoneurons innervating the dorsal muscle through synapses located in the dorsal nerve cord [32] . While the somata of both cholinergic and GABAergic motoneurons are located on the ventral side, their neural processes project to the dorsal side as circumferential commissures. In our experiments, these commissures were either severed or damaged by the glue ( Supplementary Fig. S6 ). If GABAergic PSC bursts were dependent on presynaptic inputs from cholinergic motoneurons as were cholinergic PSC bursts dependent on presynaptic inputs from command interneurons, they would be difficult to observe under the current experimental conditions. The duration and frequency of cholinergic PSC bursts are ~7 s and 3 min −1 in wild-type worms. Conceivably, the frequency and duration of cholinergic and GABAergic PSC bursts are similar in intact worms. The mean duration of cholinergic PSC bursts was comparable to that of Ca 2+ transients in body muscle cells ( Fig. 2 ), in motor neurons of semi-restrained worms [44] and in command interneurons of unrestrained worms [35] . How might the duration of PSC bursts be related with locomotion? Wild-type worms spend more than 90% of their times on forward locomotion, with the average duration of each forward movement lasting ~16 s ( [35] ), which gives ~3 forward movements per minute. The frequency of forward movements is similar to that of cholinergic PSC bursts in wild-type worms. Perhaps, one PSC burst at the NMJ corresponds to one forward movement. The rather small size of C. elegans presents a big challenge to preserve the physiological conditions of muscle cells and neurons during the gluing and dissecting processes. Over the years, we noticed that PSCs tended to display bursts in preparations with less glue application and shorter incisions. Such preparations generally showed frequent contractions of the exposed muscle cells. We used to avoid this kind of preparations or wait until the muscle contractions had waned lest that the whole-cell configuration could not be maintained. However, we later found that the whole-cell configuration could be maintained fairly easily in this kind of preparations. In the present study, we paid special attentions to minimizing the glue amount and the incision length, and finished the recording for each preparation (only from one cell) within 6–7 min. Any worms that were not properly glued and dissected were rejected before the experiment. The amount of glue used in our experiments was considerably less than that described by others [45] . As a result, our worm preparations consistently displayed PSC bursts. The persistence of PSC bursts in the head- and tail-immobilized worms suggests that PSC bursts do not rely on head or tail movements. However, PSC bursts were eliminated in worms with the head and tail cut off, suggesting that PSC bursts likely require command interneurons, which is supported by the observations that photostimulation of command interneurons can cause PSC bursts, and that command interneurons are required for rhythmic locomotion [46] . Properties of graded synaptic transmission in C. elegans have been the focus of three recent studies [5] , [6] , [7] . However, none of these studies were designed to define physiologically important endogenous PSCs. Given that the majority of nematode neurons appear to use passive propagation instead of APs [4] , [9] , [47] , PSC bursts might be used to control postsynaptic responses at many other synapses. Evoked PSCs have also been recorded from the graded synapses between inner hair cells and afferent fibres in the cochlea, and between bipolar cells and ganglion cells in the retina. The evoked responses are generally referred to as EPSCs. In cat and rat retinal ganglion cells, EPSCs evoked by light has an initial transient followed by a persistent current, from which individual PSC events could not be resolved [48] , [49] . In rat auditory afferent fibres, EPSCs evoked by hair cell depolarization with either high extracellular [K + ] or a positive voltage step appear as a burst of unitary PSC events [1] , [2] , [3] , with some of them likely representing synchronous release of multiple synaptic vesicles [50] . Some of the properties described for EPSCs at the mammalian graded synapses are reminiscent of PSC bursts at the C. elegans NMJ. C. elegans is potentially an excellent model system for investigating conserved mechanisms of graded synapses because it is amenable to powerful genetic and electrophysiological approaches. Strains and culture of C. elegans C. elegans strains used in this study were: Bristol N2 as the wild type, unc-7(e5), unc-9(fc16), EG 5182 [oxIs407(Punc-17::ChR2::mCherry lin-15(+))] [5] , EG5025 [oxIs351(Punc-47::ChR2::mCherry lin-15(+))] [5] , ZW495 [zwIs132(Pmyo-3::GCaMP2 lin-15(+))] [13] , ZW527 [zwIs132(Pmyo-3::GCaMP2 lin-15(+));slo-1(md1745)] [40] , and ZW582 [zwIs134(Pglr-1::ChR2::GFP Pmyo-2::DsRED)], ZW650 [oxIs407(Punc-17::ChR2::mCherry lin-15(+));unc-29(e1072) ], ZW651 [oxIs407(Punc-17::ChR2::mCherry lin-15(+));acr-16(ok789)], ZW652 [zwIs132(Pmyo-3::GCaMP2 lin-15(+)); zwEx173(Pglr-1::slo-1 Pmyo-2::YFP);slo-1(md1745)], ZW654 [zwIs132(Pmyo-3::GCaMP2 lin-15(+)); zwEx174(Punc-17::slo-1 Pmyo-2::YFP);slo-1(md1745)]. All worms were raised on agar plates spotted with a layer of OP50 Escherichia coli at 21 °C inside an environmental chamber. Electrophysiology All electrophysiological experiments were performed with adult hermaphrodites. The procedures for immobilizing and dissecting the worm were similar to what were described previously [24] , [38] but with special attention paid to minimizing the amount of glue application and the length of incision. Briefly, an animal was immobilized on a glass coverslip by applying Vetbond Tissue Adhesive (3M Company, St. Paul, MN). Application of the glue was generally restricted to the dorsal anterior portion (excluding the head) of the animal, allowing the head and tail to sway freely during the experiment. A short (~300 μm) longitudinal incision was made along the glued region. After clearing the viscera, the cuticle flap was folded back and glued to the coverslip, exposing several ventral body-wall muscle cells anterior to the vulva. Two representative worm preparations are shown at low and high magnifications in Supplementary Movies 6,7 , respectively. An upright microscope (FN-1, Nikon, Tokyo, Japan) equipped with a × 40 water-immersion objective (numerical aperture 0.8) was used for viewing the preparation. Borosilicate glass pipettes with a tip resistance of 3~5 MΩ were used as electrodes for current- and voltage-clamp recordings in the classical whole-cell patch clamp configuration with a Multiclamp 700B amplifier (Molecular Devices, Sunnyvale, CA), a digitizer (Digidata 1440A, Molecular Devices) and the Clampex software (version 10, Molecular Devices). Data were sampled at a rate of 10 kHz after filtering at 2 kHz. APs were recorded using the current-clamp technique without current injection whereas PSCs were recorded using the voltage-clamp technique. The holding potential was −60 mV in all the voltage-clamp experiments except for those focusing on GABAergic PSCs, which were performed at −10 mV. Ca 2+ imaging Young adult worms expressing GCaMP2 were glued and filleted for imaging spontaneous fluorescence changes of body-wall muscle cells using an electron-multiplying CCD camera (iXonEM+885, Andor Technology, Belfast, Northern Ireland), a FITC filter set (59222, Chroma Technology Corp.), a light source (Lambda XL, Sutter Instrument) and the NIS-Elements software (Nikon). Images were acquired at 16 frames per second with 10–40 ms of exposure time (no binning) for 5 min. TTL signals from the camera were used to synchronize the recordings of Ca 2+ transients and PSCs. Optogenetic stimulation Worm expressing ChR2 were grown to L4 stage on regular culture plates, and then transferred to new plates either with or without all- trans retinal 2 days before the experiment. The retinal plates were prepared by spotting each plate (60-mm diameter with 10 ml agar) with 200 μl OP50 E. coli containing 2 mM retinal (R2500, Sigma-Aldrich). Photostimulation was applied through the × 40 water-immersion objective in 2 s pulses at 30 s intervals using a light source equipped with a shutter (Lambda XL with Smart Shutter, Sutter Instrument) and a 470±20 nm excitation filter (59222, Chroma Technology Corp.). The measured light intensity at the specimen position was 6.7 mW mm −2 , which was sufficient to cause maximal evoked peak responses ( Supplementary Fig. S7 ). To analyse the correlation between the peak amplitude of evoked responses and the strength of photostimuli, laser pulses (473 nm) were produced by a solid-state laser generator (MBL-III-473, 60 mW, Changchun New Industries Optoelectronics Tech Co., Ltd, Changchun, China) with its beam aimed at the worm through an optic fibre (BFL37-200, Thorlabs, Newton, NJ) immersed in the recording solution. TTL signals from the digitizer (Digidata 1440A) were used to control the timing of optostimuli. The light intensity was measured using a power metre (PM100, Thorlabs) equipped with a standard photodiode power sensor (S121C, Thorlabs). Solutions and chemicals Two different extracellular solutions and three different pipette solutions were used, as specified in figure legends. Extracellular solution I contained (in mM) NaCl 140, KCl 5, CaCl 2 5, MgCl 2 5, dextrose 11 and HEPES 5 (pH 7.2). Extracellular solution II contained (in mM) NaCl 150, KCl 5, CaCl 2 5, MgCl 2 1, dextrose 10, sucrose 5 and HEPES 15 (pH 7.2). Pipette solution I contained (in mM) KCl 120, KOH 20, Tris 5, CaCl 2 0.25, MgCl 2 4, sucrose 36, EGTA 5 and Na 2 ATP 4 (pH 7.2). Pipette solution II contained (in mM) KCl 25, Kgluconate 115, CaCl 2 0.1, MgCl 2 5, K 4 -BAPTA 1, HEPES 10, cAMP 0.5, cGMP 0.5, Na 2 ATP 5 and Na 2 GTP 0.5 (pH 7.2). Pipette solution III contained (in mM) KCl 6.8, Kgluconate 113.2, KOH 20, Tris 5, CaCl 2 0.25, MgCl 2 4, sucrose 36, EGTA 5 and Na 2 ATP 4 (pH 7.2). (+)-TBC (T2397, Sigma-Aldrich) and gabazine (S106, Sigma-Aldrich) were dissolved in the extracellular solution to make 50 mM and 10 mM frozen stocks, respectively, and pipetted into the bath to reach their final concentrations. Data analyses Ca 2+ imaging data were analysed by assigning individual cells as separate regions of interest. The fluorescence intensities in the regions of interest over successive frames were first plotted as absolute fluorescence intensity over time using the NIS-Elements software (Nikon) and then converted to F / F 0 using the MATLAB software (The MathWorks, Inc., Natick, MA) running a custom module. Muscle cell length was measured using the NIS-Elements software, and then normalized to the maximal measured length of the cell. PSC bursts were identified as an apparent increase in PSC frequency accompanied by a baseline shift (persistent current) lasting>3 s. The boundaries of a burst were determined based on the starting and ending points of the apparent baseline shift ( Supplementary Fig. S2 ). The frequency, amplitude, charge transfer (area under the peak), half width, 10–90% rise time and decay time of PSCs were determined using MiniAnalysis (Synaptosoft, Inc., Decatur, GA). A detection threshold of 10 pA was used in initial automatic analysis, followed by visual inspections to include missed events (≥5 pA) and to exclude false events resulting from baseline fluctuations. The software was set to search for a baseline 3 ms before a PSC event and use the average of a 1-ms period as the baseline level. In a multiphasic event, the number of PSCs was determined from the apparent PSC peaks. The mean charge transfer (pC s −1 ), mean sustained current amplitude and AP frequency were measured with Clampfit software (version 10, Molecular Devices). In quantifying spontaneous PSC bursts, the extra-burst data used for comparisons were from a 10-s period (shorter if there was a preceding PSC burst) immediately before each burst. In quantifying optogenetically evoked PSCs and APs, the first three evoked responses and 10-s data immediately before each evoked response were analysed. The first 500-ms data of each evoked response were excluded from the quantification for PSC properties and sustained current amplitude to avoid complications by the large initial transient. Data graphing and statistical analyses were performed with OriginPro (version 8.5, OriginLab Corporation, Northampton, MA). Data are shown as mean±s.e. Either analysis of variance (with Bonferroni post hoc tests) or t -test (paired or unpaired) was used for statistical comparisons as specified in figure legends. P <0.05 is considered to be statistically significant. The sample size ( n ) equals the number of cells or cell pairs analysed. How to cite this article: Liu, P. et al . Postsynaptic current bursts instruct action potential firing at a graded synapse. Nat. Commun. 4:1911 doi: 10.1038/ncomms2925 (2013).